Quantitative bounds on morphodynamics and implications for reading the sedimentary record Sedimentary rocks are the archives of environmental conditions and ancient planetary surface processes that led to their formation. Reconstructions of Earth’s past surface behaviour from the physical sedimentary record remain controversial, however, in part because we lack a quantitative framework to deconvolve internal dynamics of sediment-transport systems from environmental signal preservation. Internal dynamics of landscapes—a consequence of the coupling between bed topography, sediment transport and flow dynamics (morphodynamics)—result in regular and quasiperiodic landforms that abound on the Earth and other planets. Here, using theory and a data compilation of morphodynamic landforms that span a wide range of terrestrial, marine and planetary depositional systems, we show that the advection length for settling sediment sets bounds on the scales over which internal landscape dynamics operate. These bounds provide a universal palaeohydraulic reconstruction tool on planetary surfaces and allow for quantitative identification of depositional systems that may preserve tectonic, climatic and anthropogenic signals. Landscapes are shaped by sediment-transport systems with climate, tectonics and sea level as their ultimate boundary conditions. Sedimentary strata contain a powerful record of this interplay and house information of planetary history [1] , [2] including the origin and evolution of life [3] , oxygenation of the Earth’s atmosphere [4] , global climate change [5] and the great wetting and drying of Mars [6] . Quantitative reconstructions of environmental conditions from the sedimentary record are vital, especially under present climatic changes, as they provide a pre-anthropogenic baseline to guide future landscape and climate management. Reconstructions of Earth’s past surface behaviour from the sedimentary record remain controversial [7] , [8] , [9] , however, in part because we lack a quantitative framework to deconvolve internal dynamics of sediment-transport systems from environmental signal preservation [10] , [11] , [12] . Although sedimentary deposits have been shown to contain a rich archive of environmental (allogenic) conditions and their changes [7] , [13] (that is, tectonics, climatic, sea level, anthropogenic), there is increasing recognition of the role of self-organized (autogenic) dynamics of sediment-transport systems in obscuring or even obliterating the record of externally forced environmental signals [10] , [11] , [12] , [14] . Numerical and physical experiments [10] , [11] , [12] , [14] , [15] , [16] , [17] , [18] and field investigations [8] , [19] indicate that the primary signal in physical stratigraphy can in cases be the record of the nonlinear sediment-transport dynamics, played out through geologic time. Detangling autogenic dynamics from allogenic forcing in the sedimentary record is difficult, because we lack quantitative metrics to assess where environmental conditions may be preserved in depositional archives. Crucial to solving this fundamental problem is the need to quantify the spatiotemporal scales over which autogenic dynamics manifest in fluctuations (or noise) in sediment fluxes and topography. Most autogenic dynamics in depositional landscapes are caused by coupled feedbacks between sediment-bed topography, fluid flow and sediment transport (that is, morphodynamics). The timescales of morphodynamic feedbacks can range from minutes (for example, sand ripples) to thousands of years (for example, channel avulsion on deltas) ( Fig. 1 ). The latter far exceeds historical records of sediment flux (and its variability), and therefore our understanding of the role of morphodynamic feedbacks in environmental signal preservation is based largely on small-scale physical models [10] , [15] and numerical experiments [13] , [15] , [16] , [17] , [18] . Nonetheless, upscaling results from analogue models to natural depositional systems incorporates uncertainties, and consequently, reconstructions of the sedimentary archives on both the Earth and the Mars routinely neglect any morphodynamic filtering (for example, Zhang et al. [7] ). The spatial scales of morphodynamics, on the other hand, are readily apparent in regular and periodic landforms that abound on planetary surfaces [1] ( Fig. 1 ). These landforms have yet to be synthesized in a framework that allows quantitative assessment of environmental signal preservation in the sedimentary record. 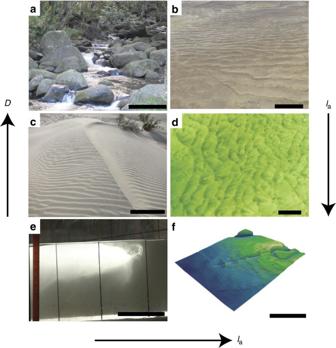Figure 1: Example morphodynamic and flow features. The advection length scale (la) increases from top to bottom with decreasing grain size (D) and left to right with increasing flow strength. (a) Step pools (1 m), (b) megaripples (Google Earth image; 500 m), (c) aeolian ripples across a larger dune (0.5 m), (d) river dunes (5 m), (e) plunging plume (0.1 m) and (f) cyclic steps (modified after Fildaniet al.39; 10 km). The numbers in the parentheses denote the scale bar dimensions. Figure 1: Example morphodynamic and flow features. The advection length scale ( l a ) increases from top to bottom with decreasing grain size ( D ) and left to right with increasing flow strength. ( a ) Step pools (1 m), ( b ) megaripples (Google Earth image; 500 m), ( c ) aeolian ripples across a larger dune (0.5 m), ( d ) river dunes (5 m), ( e ) plunging plume (0.1 m) and ( f ) cyclic steps (modified after Fildani et al. [39] ; 10 km). The numbers in the parentheses denote the scale bar dimensions. Full size image Here we first use continuity to derive an advection length scale for sediment in depositional systems and show that it may set the minimum scale over which morphodynamic interactions take place. Second, we test these ideas by comparison with a new compilation of bedform data across a wide range of terrestrial and planetary depositional environments. Third, we discuss how morphodynamic bounds can be used to divide depositional environments into three fundamental regimes characterized by different degrees of morphodynamic filtering. This new phase space has important implications for quantifying environmental signal preservation in the sedimentary record. Theoretical development To deduce the scales over which morphodynamics operate, we consider mass balance of dilute sediment transport above an evolving sediment bed that is not limited by sediment supply ( Supplementary Note 1 ). Sediment mass in transport can be treated as a phenomenon of conservation between the sediment bed, local gradients in sediment flux and the difference between vertical entrainment and settling rates of sediment [20] , [21] , [22] : Here q s is the volumetric sediment flux per unit width, λ p is the bed porosity, h is the depth of the fluid column and η is the bed elevation measured from a fixed datum. The right hand side of equation (1b) is the difference between the entrainment of sediment from the bed ( ew s ) and the near-bed settling flux of sediment ( c b w s ), where c b is the near-bed sediment concentration, w s is the settling velocity and e is a dimensionless entrainment parameter [23] , [24] . Subsidence and uplift can be neglected at the temporal scales of interest, that is, lifespans of bedforms. The local sediment flux per unit width can be written as , where q is the fluid discharge per unit width and is the depth-averaged sediment concentration, and assuming that the sediment travels at approximately the same velocity as the fluid. The sediment transport capacity per unit width can be written as , where is the depth-averaged sediment concentration at capacity. If we define (Parker et al. [25] ; Fig. 2 ), then because, where at capacity, the net deposition rate is zero and e=c b (equation (1b)). 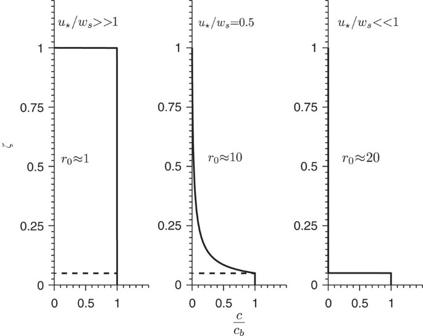Figure 2:Schematic sediment concentration profiles. These profiles were computed using the Rouse profile, wherec(ζ)is the suspended-sediment concentration at a nondimensional height ofζ=z/hfrom the bed,his the water depth,u*is the shear velocity,κ=0.41 is the von Karman constant andcbis the near-bed sediment concentration as measured at some nondimensional heightζbabove the bed (dashed line), equivalent to the bedload layer height. Three cases are shown for different values of the parameter, which partially determines the advection length scale. Substituting these definitions into equation (1b) and rearranging results in Figure 2: Schematic sediment concentration profiles . These profiles were computed using the Rouse profile , where c(ζ) is the suspended-sediment concentration at a nondimensional height of ζ = z / h from the bed, h is the water depth, u * is the shear velocity, κ =0.41 is the von Karman constant and c b is the near-bed sediment concentration as measured at some nondimensional height ζ b above the bed (dashed line), equivalent to the bedload layer height. Three cases are shown for different values of the parameter , which partially determines the advection length scale. Full size image The advection length scale, l a =uh s /w s ( Fig. 3 ), where u is the flow velocity and h s is the average settling height ( Supplementary Table 1 ), emerges as an important parameter in the sediment continuity equation. The advection length scale is the horizontal length over which an average particle is transported in the flow before falling to the bed ( Fig. 3 ). For example, if sediment is well mixed, r 0 =1 ( Fig. 2 ) and l a is the average distance travelled by a sediment particle before it settles from top of the fluid column to the bed, that is, l a =uh/w s , where h is the water depth and u is the mean horizontal velocity. For larger values of r 0 , the sediment concentration is weighted towards the bed, the effective fall height decreases (that is, h s =h/r 0 ), and therefore l a correspondingly decreases ( Figs 2 , 3 ). Although particle motions are more varied in turbulent flow than that depicted in Fig. 3 , boundary layer turbulence tends to be sufficiently isotropic such that w s remains the relevant vertical sediment velocity [26] . The above derivation is for a single sediment size, nonetheless, the concept of an advection length scale should hold in dilute depositional systems with mixed sediment sizes with each size class having a distinct advection length (for example, Lamb et al. [27] ). 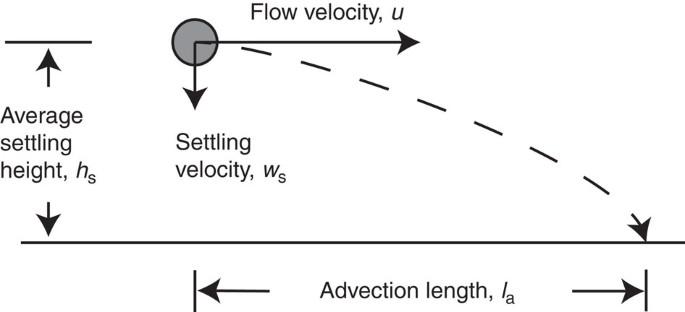Figure 3: Definition sketch of the advection length scale. The advection length scale is defined as the average horizontal distance travelled by a sediment particle before it settles to the bed (Methods,Fig. 2). Figure 3: Definition sketch of the advection length scale. The advection length scale is defined as the average horizontal distance travelled by a sediment particle before it settles to the bed (Methods, Fig. 2 ). Full size image We argue that morphodynamic feedbacks can only occur if the length scale of interest ( L ), which may be the system size for example, is larger than the advection length scale and therefore l a is herein defined as the morphodynamic microscale. The specific implication is that if l a >> L , sediment will be advected through the system before it is able to respond to topographic perturbations and local flow dynamics. This can readily be seen in the end-member limits. For example, if l a →0, the sediment flux follows the local transport capacity (equation 2) and the deposition rate follows the local gradient in transport capacity (equation 1a) [28] , [29] , a state typical of many morphodynamic bedforms. On the other hand, if l a →∞, equation (2) reduces to dq s /dx= 0 or q s =q s0 on integration (where q s0 is the sediment flux per unit width at some location upstream) and is insensitive to changes in local transport capacity. Within the aforementioned end-member limits, both advection and settling may be pertinent; however, if the length scale of the phenomenon of interest ( L ) is small compared with the advection length scale ( l a ), morphodynamic feedbacks do not occur and sediment flux is highly non-local ( q s ≈q s0 ). Previous workers have recognized the importance of the advection length scale in a variety of settings including bedform stability [30] , [31] , long-term landscape evolution [32] , turbidity currents [27] , [33] , [34] to sediment transport in turbulent flows [35] , [36] , for example. However, the novelty of our approach lies in extending its utility in placing bounds on morphodynamics, which in turn has implications for environmental signal preservation in the sedimentary record. Bounds on morphodynamics To test whether the advection length scale bounds morphodynamic interactions, we compiled a representative dataset ( Supplementary Table 1 ) on landforms and transport systems spanning a wide range in scales (10 −2 –10 6 m), sediment sizes (10 −6 –10 0 m), depositional environments (aeolian, fluvial, marine) and planets [1] (Earth, Mars, Venus) ( Figs 1 , 4 ). The advection length scale sets the minimum scale at which perturbations in fluid flow can affect bed topography due to the lag associated with settling sediment ( Fig. 3 ). Results show, across the entire dataset, that most morphodynamic landforms (blue markers in Fig. 4 ) do not exist at scales smaller than the advection length scale, thereby confirming our hypothesis that advection lengths set a minimum scale over which bedforms form. The maximum size of morphodynamic landforms also appears to scale with the advection length scale ( L ≈10 4 l a ), which may ultimately be set by the size of the depositional system [10] since large systems tend to transport fine sediment and consequently have large advection length scales. For example, the dominant scale of river deltas is set by morphodynamic feedbacks that force river avulsion at a certain spatial node [37] ; thus the largest morphodynamic feedbacks occur at the size of the delta itself ( Fig. 4 ). 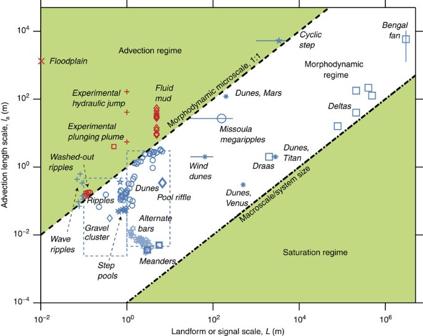Figure 4: Comparison of the advection length scale to the length scale of phenomenon of interest for a variety of systems. Morphodynamic and non-morphodynamic landforms are indicated using blue and red markers, respectively. Dashed boxes indicate bounds on the advection length scale (la) from the bedform stability diagram58(see methods;Supplementary Table 1). Because of the lack of a periodic length scale for floodplains, we chose the length scale of phenomenon of interest (L) to be negligibly small for floodplains in this plot. Figure 4: Comparison of the advection length scale to the length scale of phenomenon of interest for a variety of systems. Morphodynamic and non-morphodynamic landforms are indicated using blue and red markers, respectively. Dashed boxes indicate bounds on the advection length scale ( l a ) from the bedform stability diagram [58] (see methods; Supplementary Table 1 ). Because of the lack of a periodic length scale for floodplains, we chose the length scale of phenomenon of interest ( L ) to be negligibly small for floodplains in this plot. Full size image Classically, the Rouse parameter ( w s /, where is the shear velocity and κ is the von Karman constant of ~0.41), rather than an advection length scale, is used to determine the state of the bed with high-transport stage plane bed typically associated with substantial suspended-sediment transport [38] . The Rouse parameter scales with the advection length scale and hence, broadly, the two metrics provide similar bed-state classifications. However, anomalies highlight the important differences between these two scale parameters. For example, turbidity currents can form depositional cyclic steps on the seafloor where fine sediment is transported in suspension [39] ( Fig. 1 ; Supplementary Table 1 ). Suspended sediment, however, is not held in the flow indefinitely; like bedload sediment, it too interacts with the bed albeit over very large length scales [40] . Therefore, bed waves formed in upper plane bed regime and cyclic steps formed in fluvial and marine settings with dominantly suspended sediment are important bedforms, whereby morphodynamic feedbacks can occur, but only over kilometre scales owing to the fine sediment and large advection length scales ( Fig. 4 ). As another example, morphodynamic feedbacks in some of the largest known flows on the Earth, the Missoula outburst floods, created megaripples [41] ( Figs 1 , 4 ). Despite the coarse grains in these landforms (cobbles, boulders) that typically participate in morphodynamic feedbacks at the grain scale in most rivers (for example, gravel clusters, step pools), the flow velocities ( u ~20 m s −1 ) and depths ( h ~300 m; see Supplementary Table 1 ) of the floods were so large that morphodynamic feedbacks were limited to relatively large scales of hundreds of metres ( Fig. 4 ). Specific knowledge of the advection length scale and its correlation with the bounds on morphodynamic bedforms has implications for understanding planetary surface history. For example, given observations of sediment sizes and bedform lengths from deposits, constraints on palaeodischarge can be calculated by determining the morphodynamic microscale. Alternatively, for aeolian landforms on Mars and Titan, for example, the morphodynamic microscale can be used to predict the minimum grain sizes given information of the wind fluxes (for example, from general circulation models) and the length scales of the landforms (for example, from orbital data). Such sediment size estimates have important implications for planetary exploration, for example, on Mars where rover mobility depends on grain size of the substrate [42] . Our analysis ( Fig. 4 ) also reveals that landscape evolution and stratigraphic architecture may be substantially different in analogue experiments with advection length scales that differ from natural systems. In morphodynamic modelling, the advection length scale is ultimately the smallest scale at which coupling between the flow field and bed morphology needs to be resolved. Beyond placing bounds on morphodynamic interactions, the scaling relationship between size of bedforms and the advection length scale may have important implications for environmental signal preservation in the sedimentary record. Perturbations in fluid-flow velocity, sediment supply and land subsidence occur due to changes in land use, climate and tectonics, which create perturbations that propagate through depositional landscapes over diverse scales. We hypothesize that, in addition to sufficient accommodation and other factors recognized for long-term preservation of the sedimentary record [13] , [14] , identification of the characteristic length scales of morphodynamic feedbacks ( Fig. 4 ) allows for quantitative bounds on depositional systems that have the potential to preserve environmental perturbations of a certain scale. Here we draw on multiple examples from diverse environments to show the potential broad utility of this new framework. In the morphodynamic regime ( l a < L <10 4 l a ), internal dynamics of the depositional system are convolved with any boundary condition perturbations that manifest over the length scale L , such that the sedimentary record of these environmental signals is likely obscured or destroyed [10] . Our analysis shows that for large systems with fine sediment, morphodynamic fluctuations may span from kilometres to hundreds of kilometres, whereas in smaller systems with coarse sediment these fluctuations occur over scales ranging from centimetres to metres. Previous workers have suggested that environmental changes may only be preserved in strata if they occur at scales much larger than the scale of morphodynamics [10] . The largest morphodynamic fluctuations set the scale beyond which averaging may recover environmental signals in the depositional record; this is referred to as the saturation regime ( Fig. 4 ). For example, the deposition rate as measured from the sedimentary record in deltaic deposits is biased by stratigraphic incompleteness [8] over river-avulsion time scales [43] , which is on the order of thousands of years for large fluvial systems like the Mississippi. Thus, deltaic deposits likely record only environmental perturbations that manifest over large length scales. As another example, sedimentation rates from the Bengal fan, India, the largest submarine fan in the world, show no apparent record of the Asian monsoon intensification that lasted for ~1 Myr in the late Miocene (~8 Myr ago), but they do record changes in Himalayan tectonism that might have persisted over longer timescales [44] . Using sediment-transport velocity estimates of 1–10 m yr −1 from fan dimensions, sediment flux and sediment mass continuity (Methods), we estimate a minimum timescale associated with the saturation regime of ~0.3–3 Myr (or equivalently a saturation length of 3,000 km) for the Bengal fan. This calculation suggests that the depositional archive did not record the monsoon intensification (with equivalent length scale L ~1,000 km) because of sufficiently long morphodynamic feedbacks, which destroyed the signal ( Fig. 4 ). Although deltas and fans are often the focus of palaeoenvironmental reconstructions, our results suggest that, in the saturation regime, smaller, coarse-grained systems are likely to record allogenic forcing over a wider range in scales, potentially including anthropogenic changes. Perhaps most important is the finding of a significant range of scales in which morphodynamic fluctuations do not occur. At scales smaller than the advection length for settling sediment, referred to as the advection regime, the non-linearity associated with morphodynamic fluctuations does not exist such that we expect direct preservation of environmental signals in sedimentary strata (see equation 2), again given proper accommodation space. Thus, non-local sediment flux is a potential indicator for signal preservation in depositional systems. Figure 4 shows examples in the advection regime where morphodynamics did not develop and where the sedimentary strata faithfully recorded allogenic forcing. In the advection regime (unlike the saturation regime), it is large systems that transport fine sediment that likely record environmental signals over the largest range in scales, potentially including preservations of signals that manifest over kilometres in length [45] ( Fig. 4 ). Physical experiments provide a unique means to test signal preservation in the advection regime because, unlike field cases, both allogenic forcing and autogenic dynamics are known. For example, comparison of the advection length scale of settling sediment with plunge-point translation length from hyperpycnal plume experiments [27] ( Fig. 1 ) indicates that l a >L and the thickness and grain size of hyperpycnal-flow deposits in these experiments recorded the time history of river discharge (that is, allogenic forcing), rather than local plume dynamics. Another example is the experiments on hydraulic jumps in turbidity currents near a canyon–fan transition [46] . The computed advection length scales for the turbidity currents range from 5.5 to 165 m ( Supplementary Table 1 ), much larger than the length scale of the hydraulic jump (<1 m), which is consistent with the observation of no marked change in deposition rate in the vicinity of the hydraulic jump and consequently no record of local flow dynamics in the strata. The advection regime is dominated by landforms with planar beds and large sediment advection lengths ( Fig. 4 ), indicating that depositional environments that produce planar beds (except perhaps lower-plane bed where morphodynamic interactions at the grain scale are possible [47] ) are most likely to contain a direct record of environmental forcing—such as deep-marine basins, river floodplains and air fall. River floodplain deposits, for example, have a large advection length scale ( Fig. 4 ; Supplementary Table 1 ) and have been shown to record metrics for flood discharge on annual to decadal timescales in the absence of morphodynamic filtering [45] . The connection between signal preservation and planar beds also lends support for the often-used assumption of a direct, linear connection between orbital forcing and bed-thickness patterns in horizontally laminated strata on Mars [48] . These examples across a wide range of environments and planets demonstrate the utility of the advection length scale to define a phase space for the occurrence of morphodynamic feedbacks, which in turn helps delineate regimes where allogenic and autogenic signals can be preserved in the sedimentary record. Computation of advection length scale The advection length scale l a was computed for a variety of landforms, sediment sizes and flows from previous experimental and field studies ( Figs 1 , 2 , 3 ; Supplementary Table 1 ). This dataset is representative of a wide range of phenomena from marine to fluvial to aeolian environments on the Earth and other planets, but it is not meant to be an exhaustive compilation. The advection length scale ( l a ) was calculated using the experimental and/or field observations of the median grain size ( D 50 ) and values of flow velocity ( u ), flow depth ( h ) and vertical sediment concentration profile where reported (see Supplementary Table 1 ). Settling velocity ( w s ) was computed from grain size using the method of Dietrich [49] . In studies that did not have measurements of the vertical sediment concentration profiles, we calculated the vertical sediment concentration by assuming a Rouse profile [50] and followed the method of Smith and McLean [23] where the bedload layer height was set to 5% of the flow depth ( Fig. 2 ). Sediment velocity and advection length scale for Bengal fan The Bengal fan is the largest submarine fan on the Earth, which is about 3,000 km long and 1,000 km in width [51] . We estimated the sediment velocity scale for the Bengal fan system using sediment continuity. The modern sediment load from the Ganges–Brahmaputra river system is ~1 × 10 12 kg yr −1 (Milliman and Syvitski [52] ), of which approximately one-third is delivered to the submarine canyon–fan [53] . Assuming the bulk density of sediment (2,650 kg m −3 ) yields a sediment volume feed rate of ~1 × 10 8 m 3 yr −1 for the canyon–fan system. The width of the Bengal fan is about 1,000 km and to estimate the cross-sectional area we need a depth scale of sediment transport. We used the depth of the submarine canyon [54] , Swatch of No Ground (~1 km), as an upper bound on the depth scale of sediment transport through the system. Assuming depth scales of 10–100 m yields a sediment velocity scale of 1–10 m yr −1 . Sediment is transported in these deep, submarine canyon–fan systems by turbidity currents and our assumed depth scale agrees well with the inferred depths of turbidity currents from seismic sections in the Bengal fan [55] . The estimated sediment velocity scale, together with the length of the Bengal fan (3,000 km), yields a saturation timescale of ~0.3–3 Myr. We estimated the advection length scale ( l a ) for the Bengal fan using the modern estimates of the water discharge from the Ganges–Brahmaputra river system and the measured grain sizes accumulating on the shelf. The combined maximum annual water discharge from the Ganges–Brahmaputra river system is ~1 × 10 6 m 3 s −1 (ref. 56 ). Dividing this water discharge by the width of the submarine canyon [53] (~20 km) yields a unit water discharge of q =50 m 2 s −1 . The estimated median grain size ( D 50 =62.5–250 μm) on the inner shelf [57] yields sediment-settling velocity of 0.005–0.04 m s −1 . Since turbidity currents are the primary mode of sediment transport in the Bengal fan, we assumed a well-mixed sediment–water column ( r 0 ≈1), which yield an advection length scale of 1.3–10.4 km. How to cite this article: Ganti, V. et al. Quantitative bounds on morphodynamics and implications for reading the sedimentary record. Nat. Commun. 5:3298 doi: 10.1038/ncomms4298 (2014).